Multifunctional nanoparticles as coupled contrast agents Engineering compact imaging probes with highly integrated modalities is a key focus in bionanotechnology and will have profound impact on molecular diagnostics, imaging and therapeutics. However, combining multiple components on a nanometre scale to create new imaging modalities unavailable from individual components has proven to be challenging. In this paper, we demonstrate iron oxide and gold-coupled core-shell nanoparticles (NPs) with well-defined structural characteristics (for example, size, shell thickness and core-shell separation) and physical properties (for example, electronic, magnetic, optical, thermal and acoustic). The resulting multifunctional nanoprobes not only offer contrast for electron microscopy, magnetic resonance imaging and scattering-based imaging but, more importantly, enable a new imaging mode, magnetomotive photoacoustic imaging, with remarkable contrast enhancement compared with photoacoustic images using conventional NP contrast agents. The development of multifunctional nanoprobes enabling new imaging modalities beyond the intrinsic limitations of individual components is of considerable interest to many research areas, ranging from fundamental biology to molecular imaging and medical diagnostics. Recent advances in nanotechnology have produced various nanoparticle probes such as semiconductor quantum dots (QDs), magnetic nanoparticles (MNPs) and metallic NPs. Their unique electronic, magnetic, optical and structural properties have addressed a broad spectrum of biomedical applications, such as ultrasensitive detection, medical imaging and targeted therapeutics [1] , [2] , [3] . Similar to conventional small molecule-based imaging probes, however, each type of nanoprobe displays distinct advantages and limitations [4] , [5] . For example, MNPs have become an important contrast agent in T2-weighted magnetic resonance imaging (MRI) because MRI offers high resolution and excellent tissue penetration depth. On the other hand, MRI is not as sensitive as optical imaging or positron emission tomography, and is difficult to visualize in microscopic tissue examination [6] . Similarly, gold NPs are often used in scattering-based imaging and offer high sensitivity, high resolution and multiplexing capability [7] . However, the tissue penetration depth of optical imaging is limited to millimetres [6] . Therefore, a major challenge is how to engineer molecular probes with integrated functionalities while still maintaining compact sizes [8] . Furthermore, it is highly desirable that nanoprobes with coupled functionalities will enable new imaging modes not available from each individual component for enhanced contrast specificity. A long sought-after coupled imaging probe is noble metal, such as platinum and gold, -coated MNPs [9] , [10] , with precisely controlled shell thickness and smooth surface, because of a number of desirable properties, including magnetic attraction, near-infrared (NIR) absorption, photon scattering and easy biomolecular conjugation through stable thiolate–gold interaction. Several attempts have been made by directly coating gold onto MNPs [11] , [12] , [13] , [14] , [15] , [16] , [17] , [18] or MNP-silica composites (using the low dielectric permittivity of silica) [19] , [20] , [21] . However, neither approach simultaneously produces NPs with NIR response (critical for in vivo imaging and therapy) and yet maintains compact particle size (affects tissue penetration and plasma circulation). For example, gold coating on MNP-silica composites often results in large particles of 100–200 nm in diameter with uneven surfaces [19] , [20] , [21] . Similarly, direct coating of gold onto iron oxide NPs requires both a large core particle and thick gold coating for NIR response [12] , [13] , [14] . This is because, in contrast to silica–gold core-shell NPs, the absorption profile of which red-shifts with decreasing shell thickness, iron oxide–gold core-shell particles absorb at longer wavelengths with increasing shell thickness [13] . As a consequence, compact MNPs with thin gold coating only absorb in the visible spectrum [17] , [18] . For NIR response, MNP-gold core-shell particles must be large in overall size (100–400 nm) [12] , [13] , [14] . Here, we report a new generation of compact, uniform, NIR-responsive MNP-gold core-shell nanostructures by creating a gap between the core and the shell. Not only does this approach produce a magnetically sensitive NP with both strong NIR and MRI responses, it also enables a new modality, magnetomotive photoacoustic (mmPA) imaging. Compared with PA imaging using conventional metallic NPs, mmPA imaging with a coupled agent provides the same sensitivity but with markedly improved contrast specificity. Indeed, all PA signals not created by the coupled NPs can be potentially suppressed to the electronic noise limit of the imaging system. 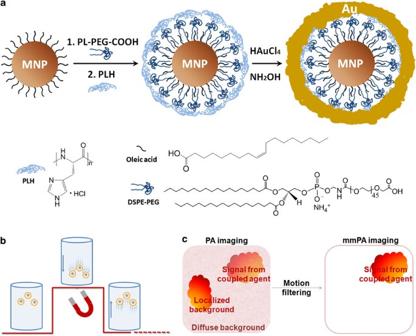Figure 1: Schematic of MNP-gold core-shell NPs and mechanism of background suppression using mmPA. (a) Key steps involved in hybrid NP synthesis (figure not drawn to scale). Monodisperse hydrophobic MNPs coated with oleic acids are first solubilized using amphiphilic PL-PEG-COOH. PLH, which is capable of chelating metal ions, is then adsorbed onto PL-PEG-COOH by electrostatic interaction. On addition of gold ions and a reducing reagent, thin gold shells form on the polypeptide template rather than directly on core nanoparticles. The molecular structures of oleic acid, PL-PEG-COOH and PLH are shown below the reaction scheme. (b) Schematic of MNP-gold core-shell NPs' response to a magnetic field. The underlying red curve represents field strength. The coupled agents move as the magnetic field is turned on and off. (c) Schematic of contrast enhancement in mmPA imaging. mmPA imaging suppresses regions not susceptible to a controlled magnetic field while identifying regions with coupled agents responsive to a magnetic field. Synthesis of MNP-gold core-shell NPs Figure 1 schematically illustrates the major steps in producing MNP-gold-coupled NPs and the manner in which they can be used for mmPA imaging. Highly monodispersed MNPs with hydrophobic surface ligands, oleic acid, are first solubilized into an aqueous solution using phospholipid-polyethylene glycol terminated with carboxylic acid (PL-PEG-COOH). The hydrophobic PL segment interdigitates with oleic acids through hydrophobic interactions, whereas the PEG block facing outwards renders MNPs water-soluble and negatively charged because of the terminal carboxylic acids. To create anchor points for gold shell growth, a layer of positively charged peptide, poly- L -histidine (PLH), is adsorbed onto the outer surface of MNP-PEG through charge–charge interaction at pH 5–6. Indeed, zeta potentials of the PEG-solubilized MNPs before and after coating with PLH were −15.5 and +9.1 mV, respectively. This surface charge inversion suggests a successful layer-by-layer surface coating of polyelectrolytes (ionic polymers) on NP surfaces. Figure 1: Schematic of MNP-gold core-shell NPs and mechanism of background suppression using mmPA. ( a ) Key steps involved in hybrid NP synthesis (figure not drawn to scale). Monodisperse hydrophobic MNPs coated with oleic acids are first solubilized using amphiphilic PL-PEG-COOH. PLH, which is capable of chelating metal ions, is then adsorbed onto PL-PEG-COOH by electrostatic interaction. On addition of gold ions and a reducing reagent, thin gold shells form on the polypeptide template rather than directly on core nanoparticles. The molecular structures of oleic acid, PL-PEG-COOH and PLH are shown below the reaction scheme. ( b ) Schematic of MNP-gold core-shell NPs' response to a magnetic field. The underlying red curve represents field strength. The coupled agents move as the magnetic field is turned on and off. ( c ) Schematic of contrast enhancement in mmPA imaging. mmPA imaging suppresses regions not susceptible to a controlled magnetic field while identifying regions with coupled agents responsive to a magnetic field. Full size image Previously, we synthesized QD-gold core-shell particles using similar approaches and showed that, in contrast to commonly used primary amines, the imidazole groups in PLH are capable of immobilizing Au 3+ ions on QD surfaces at high packing density [22] . This is perhaps not surprising as metal ion chelating by histidine-containing peptides has been studied extensively for affinity chromatography. The multilayer organic molecules coated on the MNP surface (oleic acid, PL-PEG and PLH) function as an effective barrier preventing gold ions from direct growth on the iron oxide core. Further reduction of Au 3+ with a reducing reagent leads to the formation of multifunctional MNP-gold core-shell particles with clear separation and only a small size increase over the original MNPs. In contrast to the QD-gold hybrid, which does not offer new imaging mechanisms [22] , the resulting coupled MNP-gold nanoprobe provides contrast not only for conventional modalities such as transmission electron microscope (TEM), optical imaging, PA imaging and MRI but also for the new modality of mmPA imaging. Principle of mmPA imaging Figure 1b illustrates how MNP-gold NPs can be manipulated for mmPA imaging. During real-time PA data acquisition, a pulsed magnetic field is applied. Voxels within the imaging region experience a force induced by the local field and magnetization. When the field is on, MNP-gold NPs move as a result of their strong magnetization, creating a moving source within a PA image. When the field is turned off, MNP-gold NPs return to their original positions. Non-magnetic PA sources do not move coherently with the applied field during this entire interval. Consequently, coherent motion processing of a PA image sequence ( Fig. 1c ) can identify sources related to MNP-gold NPs and reject all background signals, whether from diffuse or localized sources. Such processing can greatly enhance the contrast specificity of the NP. By comparison, bare MNPs are not a suitable contrast agent for PA or mmPA imaging, even though they can respond to magnetic field. Bare MNPs do not absorb efficiently in the NIR and, consequently, exhibit poor PA efficiency. Similarly, although plasmonic nanomaterials, such as Au nanorods, have large NIR absorption per particle and high PA efficiency, their signals could be buried by high backgrounds often seen in optical and acoustic imaging. Characterization of MNP-gold-coupled contrast agents Although the engineering of MNP-gold NPs applies to MNPs of various sizes ( Supplementary Fig. S1 ), the synthesis, characterization and applications of the coupled nanoprobe discussed below are focused on one representative MNP with a 25 nm diameter ( Fig. 2a ). TEM images show MNP-gold core-shell NPs with different shell thickness and a gap of ~3 nm between core and shell due to the low electron density of the embedded organic molecules. In contrast to conventional approaches in which only thick gold nanoshells can be coated onto NPs [23] , PLH-templated gold deposition can be controlled with nanometre precision to form an ultrathin and relatively smooth shell layer [22] . As a result, a gold nanoshell less than 3–4 nm thick enabled direct observation of the internal structure of the MNP-gold core-shell NPs ( Fig. 2b,c ). When the shell thickness was slightly increased to 4–5 nm, the core-shell internal structure disappeared and manifested as solid dark dots ( Fig. 2d ). Note that the 4–5 nm shell thickness was not directly measured (not visible under TEM), but was derived from the overall particle size increase compared with original MNPs and MNPs coated with thin gold layers ( Fig. 2e–h ). 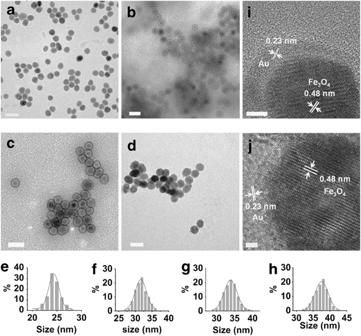Figure 2: TEM imaging of the MNP-gold-coupled agents. (a–d) TEM images and (e–h) size distribution histograms of (a) PL-PEG-COOH/PLH-coated MNPs (polymer layer not visible under TEM because of low electron density), and (b–d) MNP-gold core-shell NPs with various shell thickness (b, ~1 to 2 nm;c, 2–3 nm;d, 4–5 nm). Scale bars are 50 nm. (e–h) The particle size histograms are plotted from analysis of >150 particles for each sample. Mean and s.d. for the various distributions are, respectively, 24.4 and 1.3 nm in panele; 31.7 and 2.5 nm in panelf; 33.9 and 1.9 nm in panelg; and 37.4 and 2.0 nm in panelh. (i–j) Representative high-resolution-TEM images of MNP-gold core-shell NPs with shell thickness of ~2 to 3 nm. The lattice spacing of the MNP core measures at 0.48 nm corresponding to the (111) plane of Fe3O4, whereas the (111) plane of face-centred cubic (fcc) Au shows 0.23 nm lattice spacing. The scale bar is 5 nm for paneliand 2 nm for panelj. Figure 2: TEM imaging of the MNP-gold-coupled agents. ( a – d ) TEM images and ( e – h ) size distribution histograms of ( a ) PL-PEG-COOH/PLH-coated MNPs (polymer layer not visible under TEM because of low electron density), and ( b – d ) MNP-gold core-shell NPs with various shell thickness ( b , ~1 to 2 nm; c , 2–3 nm; d , 4–5 nm). Scale bars are 50 nm. ( e – h ) The particle size histograms are plotted from analysis of >150 particles for each sample. Mean and s.d. for the various distributions are, respectively, 24.4 and 1.3 nm in panel e ; 31.7 and 2.5 nm in panel f ; 33.9 and 1.9 nm in panel g ; and 37.4 and 2.0 nm in panel h . ( i – j ) Representative high-resolution-TEM images of MNP-gold core-shell NPs with shell thickness of ~2 to 3 nm. The lattice spacing of the MNP core measures at 0.48 nm corresponding to the (111) plane of Fe 3 O 4 , whereas the (111) plane of face-centred cubic (fcc) Au shows 0.23 nm lattice spacing. The scale bar is 5 nm for panel i and 2 nm for panel j . Full size image Given that TEM imaging under inappropriate focusing conditions could possibly show blurred ring structures around NPs, high-resolution TEM was also performed to ensure that the core-shell structure observed was not an imaging artefact. Two representative images are shown in Figure 2i,j . Despite their relatively low contrast compared with low-magnification images on ultrathin nanomaterials [24] , the signature crystal lattices of iron oxide and gold are clearly visible, which unambiguously confirms the core-shell structure. We also noted that, because of the ultrathin nature, it would be difficult to achieve a completely uniform gold shell without gaps or pores. Previous research has shown that, although gold shells impart remarkable resistance to oxidation and acid-etching for embedded iron oxide NPs, a relatively thick Au layer is needed to completely isolate the core particle from the environment [11] , [15] . Further improvements in the evenness of thin shells could be made by new nanocrystal synthesis techniques such as non-epitaxial shell growth [25] . Nevertheless, for this paper, the most desirable property is not a poreless shell, but strong NIR absorption. Next, we thoroughly characterized the optical and magnetic properties of hybrid NPs, as well as their stability against NIR laser irradiation. Core-shell NPs display shell-type NIR absorption [23] . 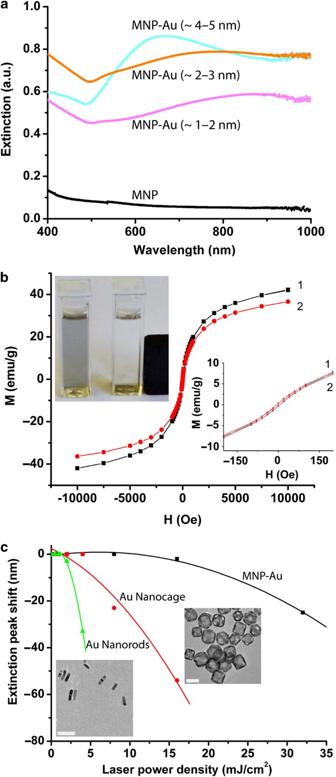Figure 3: Optical and magnetic properties and stability of the MNP-gold hybrid NPs. (a) Extinction spectra of MNPs successively coated with PL-PEG-COOH and PLH (black), and with gold nanoshells of various thickness, 1–2 nm (purple), 2–3 nm (orange) and 4–5 nm (blue). As the gold nanoshell thickness increases, the spectral intensity increases and the peak centre blue-shifts. (b) Magnetization as a function of magnetic field at room temperature for MNP (black) and MNP-gold (2–3 nm shell thickness) (red). The gold shell coating has negligible effect on the magnetic behaviour of MNPs. Insets show the absence of magnetic hysteresis and magnetic separation of MNP-gold NPs. (c) Photothermal stability of MNP-gold NPs in comparison with gold nanocages and nanorods. Extinction peak shifts as a function of laser fluence indicate that nanocages and nanorods start to quickly degrade at 5 mJ cm−2, whereas MNP-gold hybrid NPs remain stable against laser irradiation of approximately three times higher fluence. TEM images of nanocages and nanorods are shown as insets, scale bars are 50 nm. Figure 3a shows the extinction spectra of MNP-gold core-shell hybrid particles corresponding to the TEM images shown in Figure 2a–d . Compared with MNPs successively coated with PL-PEG-COOH and PLH polymer layers exhibiting negligible NIR absorption, the surface plasmon resonance (SPR) band appeared in the NIR spectrum with formation of thin gold nanoshells. The SPR peaks of the core-shell structures are significantly enhanced (intensity well above that of the original MNP core), which is desirable for PA imaging. Note that the elevated curves are part of the extinction signals, instead of noise, which is commonly seen in shell-type plasmonic materials [23] . For 1- to 2-nm-thick gold shells, the SPR band centred around 900 nm. As the thickness increased to 2–3 and 4–5 nm, the SPR extinction peak blue-shifted to 760 and 660 nm, respectively, following a trend similar to that of silica–gold nanoshells [23] . This spectroscopic measurement confirms the electron microscopy results of Fig. 2, showing that the gold shell is separated from the iron oxide core (red-shift in the visible spectrum with increasing shell thickness would be expected otherwise [13] ). We also noticed that the extinction peaks of hybrid NPs are broader than theoretical values. Such line broadening is commonly seen in virtually all gold shell nanostructures [13] , [14] , [17] , [26] , [27] , and has been attributed to the combination of a number of factors including phase-retardation effects, size distribution of both cores and shells and electron scattering at shell interfaces [28] . Figure 3: Optical and magnetic properties and stability of the MNP-gold hybrid NPs. ( a ) Extinction spectra of MNPs successively coated with PL-PEG-COOH and PLH (black), and with gold nanoshells of various thickness, 1–2 nm (purple), 2–3 nm (orange) and 4–5 nm (blue). As the gold nanoshell thickness increases, the spectral intensity increases and the peak centre blue-shifts. ( b ) Magnetization as a function of magnetic field at room temperature for MNP (black) and MNP-gold (2–3 nm shell thickness) (red). The gold shell coating has negligible effect on the magnetic behaviour of MNPs. Insets show the absence of magnetic hysteresis and magnetic separation of MNP-gold NPs. ( c ) Photothermal stability of MNP-gold NPs in comparison with gold nanocages and nanorods. Extinction peak shifts as a function of laser fluence indicate that nanocages and nanorods start to quickly degrade at 5 mJ cm −2 , whereas MNP-gold hybrid NPs remain stable against laser irradiation of approximately three times higher fluence. TEM images of nanocages and nanorods are shown as insets, scale bars are 50 nm. Full size image The magnetization of hybrid NPs (2–3 nm gold shell) was measured using superconducting quantum interference device (SQUID) magnetometry. The temperature dependence of the zero-field-cooled/field-cooled magnetization is shown in Supplementary Figure S2 . The two curves overlap at high temperature and quickly depart from each other as the temperature decreases. The zero-field-cooled curves show maxima at 275 and 270 K (blocking temperature, T b ) for MNPs before and after coating with thin Au shells, which is characteristic of superparamagnetism [9] , [20] . The T b values of MNPs are well below room temperature and the slight decrease after surface coating has been previously observed as well. It is believed to reflect the decreased coupling of the magnetic moments as a result of the increased interparticle spacing of magnetic cores [18] , which is due to a combination of Au and polymer capping shells for the hybrid NPs. For superparamagnetic colloids, the M–H curve should not show hysteresis when measured above T b . Indeed, no hysteresis was detected at room temperature after MNPs were coated with a thin gold shell and the saturation magnetization of magnetic cores was only reduced slightly ( Fig. 3b ). The compact core-shell NPs do not aggregate in solution, but respond magnetically. When an external magnetic field was applied, NPs were slowly isolated by the magnetic force (>3 h). The remaining liquid became colourless, indicating that the plasmonic response was indeed due to gold nanoshells on MNPs instead of self-nucleated gold NPs ( Fig. 3b inset). Besides optical and magnetic properties, we further characterized particle stability under NIR laser irradiation, as the biomedical applicability of this technology strongly depends on probe stability. For example, one of the most common uses of plasmonic nanomaterials is photothermal therapy, in which electromagnetic radiation is converted into heat to treat diseased cells [7] , [29] . Therefore, nanoprobe stability is directly linked with therapeutic effects. Compared with two popular gold-based NIR-responsive nanoprobes, nanorods and nanocages [30] , [31] , [32] , [33] , [34] , both of which have been used in imaging and therapy, MNP-gold core-shell NPs exhibited remarkable stability under identical laser irradiation. As shown in Figure 3c , both gold nanorods and nanocages were stable at laser fluences below 2 and 6 mJ cm −2 , respectively. Above these fluences, significant SPR peak shifts were observed indicating nanoprobe degradation. In contrast, only slight peak shifts were observed for MNP-gold hybrid NPs when the laser fluence was increased to 10–15 mJ cm −2 . Significant spectral shifts were also observed when the laser fluence was further increased. Multimodality imaging using coupled contrast agents To demonstrate the use of this technology for multimodality imaging, we first tested MNP-gold hybrid NPs with conventional modalities, including dark field, PA and MR imaging. In addition to the EM images shown in Figure 2 , based on the high electron density of both core and shell materials, MNP and gold have highly complementary features for other imaging modes. 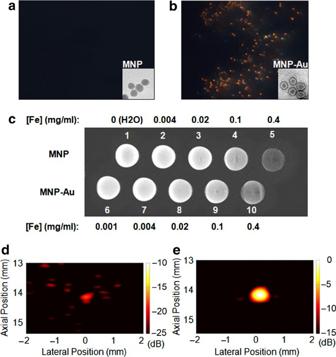Figure 4: Multimodality imaging using MNP-gold hybrid NPs. (a,b) Dark-field imaging of single MNPs spread on glass coverslips before and after gold nanoshell coating. The coated MNPs are readily detectable under current experimental conditions (insets show corresponding TEM images). (c) T2-weighted MR images of bare and gold-coated MNPs at various dilutions. Signal strength is indicated by the darkness of the images. At the same concentrations, the MRIs are indistinguishable between the two series, indicating unchanged magnetic properties before and after gold nanoshell coating. (d,e) Cross-sectional PA images of a tube filled with (d) 5 nM MNPs and (e) 5 nM MNP-gold NPs on a dB scale. A level of 0 dB corresponds to the maximum signal level among both images. Note that a different dynamic range was used for better visualization. Signal-to-noise ratio can be improved by 1 order of magnitude (20 dB) when MNP-gold NPs are used. As shown in Figure 4a,b , the strong scattering property of gold nanoshell makes the hybrid NPs an excellent optical imaging probe. Samples of dilute uncoated and gold shell-encapsulated MNPs were spread on glass coverslips, resulting in spatially isolated single NPs on the surface. Under dark field imaging conditions, MNP-gold hybrid NPs are easily detectable but not the original MNPs. On the other hand, scattering-based imaging does not allow deep tissue imaging, but MRI does. To demonstrate the MRI capability of these hybrid particles, we compared them with conventional MNPs. Serial dilutions of MNPs with and without gold nanoshell coating exhibited nearly identical image contrast ( Fig. 4c ), which confirmed the SQUID results that showed that MNPs maintained their magnetic properties after being coated with thin gold shells. Figure 4: Multimodality imaging using MNP-gold hybrid NPs. ( a , b ) Dark-field imaging of single MNPs spread on glass coverslips before and after gold nanoshell coating. The coated MNPs are readily detectable under current experimental conditions (insets show corresponding TEM images). ( c ) T2-weighted MR images of bare and gold-coated MNPs at various dilutions. Signal strength is indicated by the darkness of the images. At the same concentrations, the MRIs are indistinguishable between the two series, indicating unchanged magnetic properties before and after gold nanoshell coating. ( d , e ) Cross-sectional PA images of a tube filled with ( d ) 5 nM MNPs and ( e ) 5 nM MNP-gold NPs on a dB scale. A level of 0 dB corresponds to the maximum signal level among both images. Note that a different dynamic range was used for better visualization. Signal-to-noise ratio can be improved by 1 order of magnitude (20 dB) when MNP-gold NPs are used. Full size image Besides scattering, the second feature unique to the gold nanoshell is strong NIR absorption, and companion energy release in the form of heat, which can be used for photothermal therapy [35] and PA imaging [36] , [37] . Compared with the shallow photon penetration depth of scattering techniques, PA imaging can sample optical phenomena within tissue to a depth of several centimetres [38] . It is also much cheaper to operate and more portable than MRI. Absorption of pulsed NIR laser light creates acoustic sources within tissue, wherein the source strength is proportional to the local absorption of the optical pulse. An image is formed using conventional ultrasound technology, in which PA contrast is directly related to optical absorption. To test the efficacy of MNP-gold particles as PA contrast agents, water solutions consisting of no particle, 5 nM MNPs and 5 nM MNP-gold hybrid NPs were injected sequentially into a polycarbonate tube and illuminated with a 750 nm pulsed laser. Figure 4d,e shows cross-sectional PA images of the tube corresponding to the different solutions on a decibel (dB) scale, with 0 dB corresponding to the maximum signal level across all images. Compared with the MNP solution, MNP-gold of the same concentration improved the image signal-to-noise ratio by nearly 1 order of magnitude (that is, 20 dB) because of the strong gold-shell SPR absorption. mmPA using MNP-gold-coupled contrast agents Next, we demonstrated that MNP-gold hybrid NPs' strong magnetization and NIR absorption enable mmPA imaging with significantly improved contrast specificity compared with conventional PA imaging. A 3-mm-thick, 10% polyvinyl alcohol (PVA) disk was constructed as an imaging phantom. It contained three 2-mm-diameter cylindrical inclusions made of 10% PVA mixed with 8% 15-μm polymer beads. The first, containing gold nanorods with absorption comparable to that of 3 nM MNP-gold hybrid NPs, serves as a magnetic reference, that is, a localized 'background' region to be suppressed in mmPA imaging; the second, containing 3 nM MNP-gold hybrid NPs, serves as an object of interest; and the third, containing 3 nM MNPs, serves as an optical reference. An electromagnet generating 5-s 0.7-Tesla pulses was placed under a water tank holding the phantom. 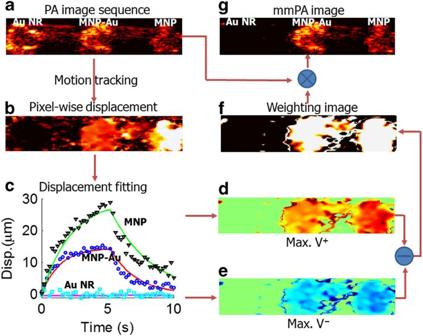Figure 5: Data processing in mmPA imaging of MNP-gold hybrid NPs. A PVA phantom holds three 2-mm-diameter inclusions, in which the one on the left contains gold nanorods with absorption comparable to the 3 nM MNP-gold hybrid NPs placed in the centre inclusion, and the third inclusion on the right contains 3 nM MNPs. A conventional PA image of this phantom is presented in (a) on a logarithmic scale over a 40 dB display range. The gold nanorod inclusion on the left serves as a magnetic reference and mimics strong background tissue signals. The MNP inclusion on the right serves as an optical reference to MNP-gold hybrid NPs. Using a sequence of PA images acquired while a magnetic field was turned on and then off over a 10-s interval, the maximum displacement resulting from the action of the magnetic field is presented in (b) on a pixel–pixel basis over a display range of (0 (dark), 30 (light)) μm. (c) Three representative displacement traces and their fitted curves over the entire time interval of the experiment for pixels in different inclusions. Using these curves, velocity was computed over the full 10-s interval and the maximum positive and negative velocities, presented in (d) and (e) over a (−20, 20) μm s−1display range, were used to create a weighting image, presented in (f) over a (0, 1) display range, based on the magnitude of difference between peak positive velocity in the first half and peak negative velocity in the second half. (g) mmPA image produced from the product of (a) with (f) over a 40 dB display range demonstrates that the gold nanorod inclusion mimicking a strong background signal is almost completely suppressed. Figure 5a shows a cross-sectional PA image on a dB scale of the PVA phantom at 720 nm optical wavelength, with 0 dB corresponding to the maximum signal level across all images. The inclusion with MNP-gold hybrid NPs (middle) is one order of magnitude (that is, 20 dB) brighter than the one with MNPs (right), in agreement with Fig. 3d,e . Although the inclusion with gold nanorods (left) has PA strength comparable to that with MNP-gold hybrid NPs, it is suppressed in the mmPA image shown in Figure 5g . Figure 5: Data processing in mmPA imaging of MNP-gold hybrid NPs. A PVA phantom holds three 2-mm-diameter inclusions, in which the one on the left contains gold nanorods with absorption comparable to the 3 nM MNP-gold hybrid NPs placed in the centre inclusion, and the third inclusion on the right contains 3 nM MNPs. A conventional PA image of this phantom is presented in ( a ) on a logarithmic scale over a 40 dB display range. The gold nanorod inclusion on the left serves as a magnetic reference and mimics strong background tissue signals. The MNP inclusion on the right serves as an optical reference to MNP-gold hybrid NPs. Using a sequence of PA images acquired while a magnetic field was turned on and then off over a 10-s interval, the maximum displacement resulting from the action of the magnetic field is presented in ( b ) on a pixel–pixel basis over a display range of (0 (dark), 30 (light)) μm. ( c ) Three representative displacement traces and their fitted curves over the entire time interval of the experiment for pixels in different inclusions. Using these curves, velocity was computed over the full 10-s interval and the maximum positive and negative velocities, presented in ( d ) and ( e ) over a (−20, 20) μm s −1 display range, were used to create a weighting image, presented in ( f ) over a (0, 1) display range, based on the magnitude of difference between peak positive velocity in the first half and peak negative velocity in the second half. ( g ) mmPA image produced from the product of ( a ) with ( f ) over a 40 dB display range demonstrates that the gold nanorod inclusion mimicking a strong background signal is almost completely suppressed. Full size image An mmPA image can be derived from a series of PA images in various ways. Figure 5 illustrates the current signal processing scheme. A conventional PA image ( Fig. 5a ) sequence was acquired in synchrony with a magnetic pulse. The displacement of each pixel in a PA image from its initial position was tracked using a conventional speckle tracking algorithm [39] over the entire 10-s interval, with the magnetic pulse spanning the first 5 s. Figure 5b shows the maximum displacement at the end of the magnetic pulse. For each pixel, we fitted the displacement as linear functions of time over the two 5-s intervals when the field was on/off. A pixel with positive slope in the first half and negative slope in the second half was subsequently fitted to two cascaded exponential functions using nonlinear least squares curve fitting. Three representative fitted curves are shown in Figure 5c for three pixels within the inclusions. Using these curves at every pixel, velocity was computed over the full 10-s interval ( Supplementary Movie S1 ), and the maximum positive and negative velocities, shown in Figure 5d,e , were used to create a weighting image ( Fig. 5f ) on the basis of the magnitude of difference between the peak positive velocity in the first half and the peak negative velocity in the second half. Figure 5g shows the mmPA image produced from the product of Fig. 5a,f , in which the gold nanorod inclusion is almost completely suppressed. Although the principle of suppressing strong PA sources not susceptible to an applied magnetic field (for example, the gold nanorod inclusion above) in mmPA imaging has been demonstrated, finite background motion in real clinical imaging from physiological sources such as cardiac motion and respiration can interfere with induced motion. Other imaging modalities, such as acoustic radiation force impulse imaging and thermal strain imaging, have a similar problem of tracking small induced displacements during physiological motion. Robust signal processing methods have been developed to track induced motion by synchronizing the data acquisition sequence with physiological motion [40] , [41] . Similar methods can be developed for clinical applications of mmPA imaging [42] . We also note that motion filtering may not need to be performed for all PA imaging for contrast enhancement, but high background is commonly seen in PA imaging similar to optical imaging and MRI. In mmPA imaging, the induced motion depends not only on the magnetic field but also on tissue elastic properties. Therefore, in biomedical applications, it is hard to quantify the contrast agent concentration on the basis of motion alone. For example, displacements and velocities in the MNP inclusion were slightly greater than those in the MNP-gold hybrid NP inclusion, primarily because of differences in the elasticity of inclusions ( Supplementary Fig. S3 ). However, the induced motion, regardless of scale, is coherent with the applied magnetic field. By detecting motion in response to a time-varying magnetic field, contrast can be greatly improved. The ability to enhance regions with targeted contrast agents makes mmPA imaging an attractive modality for molecular diagnostics. In addition, because the displacement time course depends on tissue elastic properties (for example, after the magnetic field is turned off, displaced tissue moves back to its original position subject only to intrinsic elastic properties such as relaxation), mmPA imaging can potentially also be used for elasticity imaging. In conclusion, a new class of iron oxide–gold core-shell NPs has been developed. In contrast to previous arts in which gold shells are deposited directly on iron oxide or iron oxide–silica composites, the core and shell of our particles are spatially separated with a dielectric polymer layer. This method allows the formation of uniform MNP-gold particles that are simultaneously compact in size and responsive in the NIR spectrum, which has not been achieved previously. The resulting NPs show highly integrated properties, including electronic, magnetic, optical, acoustic and thermal responses, which allow multimodality imaging. Beyond conventional NP-based imaging modalities such as TEM, optical imaging, MRI and PA, coupling of magnetic motion with photothermal conversion enables mmPA, a new modality with remarkable contrast enhancement compared with conventional PA imaging. We envision that the gold surface will also allow simple conjugation with biomolecular targeting ligands to develop all-in-one nanostructures for non-invasive imaging, molecular diagnosis and hyperthermia-based treatment of complex diseases. Chemicals and instruments Unless specified, chemicals were purchased from Sigma-Aldrich and used without further purification. Oleic acid-capped monodisperse superparamagnetic iron oxide nanocrystals of different sizes were a gift from Oceannanotech LLC. PL-PEG-COOH (DSPE-PEG 2000 carboxylic acid) was purchased from Avanti polar lipids. PLH (MW ≥5,000) was used as the templates to direct gold nucleation and growth. A UV-2450 spectrophotometer (Shimadzu) was used to characterize NP absorption spectra. A tabletop ultracentrifuge (Beckman TL120) was used for NP purification and isolation. Particle size was measured on a CM100 TEM (Philips EO). Dark field images were obtained on an IX-71 inverted microscope (Olympus) equipped with a Q-color5 digital colour camera (Olympus). SQUID magnetometry was measured at 300K on a Quantum Design MPMS-5S SQUID Magnetometer (Quantum Design). Solubilization of MNPs with PL-PEG-COOH Oleic acid-coated MNPs (1 mg) and PL-PEG-COOH (1.4 mg) were mixed in chloroform (1 ml), followed by slow evaporation of the solvent. The residual solid was heated to 80°C for 5 min to completely removed chloroform. The MNPs became soluble after adding deionized (DI) water (1 ml) and brief sonication. Excess lipids were purified from solubilized MNPs with repeated ultracentrifugation (25,000 r.p.m. for 1 h×3 times). The purified MNPs were redispersed in 4 ml of DI water, to which 1.1 mg of PLH was added. The pH of the solution was adjusted to 5–6 using 0.1 N HCl. After incubation for 60 min, MNPs coated with PLH were again purified with ultracentrifugation and dispersed in 5 ml of DI water. Gold nanoshell growth A volume of 890 μl of DI water and 10 μl of HAuCl 4 (w/w 1%) aqueous solution (pH adjusted to 9–10 with NaOH) were added to 100 μl of MNP–PLH solution, and incubated for 20 min. A reducing agent NH 2 OH·HCL (20 mM, 20 μl) was then introduced to initiate the surface-confined Au shell growth. On mixing, the colloidal solution changed colour from brownish-black to dark blue over a few minutes, indicating the formation of gold nanoshells. The resultant gold shells are typically ~2 to 3 nm in thickness, which can be facilely tuned by changing the amount of gold ions. After synthesis, PEG-SH was used to enhance colloidal stability. Photoacoustic imaging Particle samples were injected into a polycarbonate tube (CTPC167-200-5, Paradigm Optics; 167 and 200 μm inner and outer diameters, respectively). A frequency-doubled YAG pulsed laser (Surelite I-20, Continuum) with 5-ns pulse width pumped an optical parametric oscillator (Surelite OPO Plus, Continuum) to illuminate the tube at 750 nm wavelength and 3.3 mJ cm −2 fluence. PA signals were received by the central 32 elements of an ultrasound linear array (L 14-5/38, Ultrasonix, Burnaby) and recorded by an ultrasound scanner (Sonix RP, Ultrasonix). A delay-and-sum beamforming algorithm was used for image reconstruction. For NP stability against laser irradiation, samples were subjected to 30 min of continuous irradiation at wavelengths close to the SPR peaks of each particle sample at fixed laser fluence. Magnetomotive photoacoustic imaging A phantom of 10% PVA disk of 3-mm thickness was constructed using three short freeze–thaw cycles. Three 2-mm-diameter cylindrical inclusions made of 10% PVA mixed with 8% 15-μm polymer beads (Bangs Laboratories) were placed within the phantom: the first one contained gold nanorods with about the same absorption coefficient as 3 nM MNP-gold hybrid NPs, the second contained 3 nM MNP-gold hybrid NPs and the third contained 3 nM MNPs. An electromagnet integrated with a DC power amplifier, a current amplifier and a function generator (Agilent 33250A), producing 5-s 0.7-Tesla pulses, was placed under a water tank holding the phantom. A frequency-doubled YAG pulsed laser (Surelite I-20, Continuum) with 5-ns pulse width pumped an optical parametric oscillator (Surelite OPO Plus, Continuum) to illuminate the PVA phantom at 720 nm wavelength and 2.3 mJ cm −2 fluence. A 15-MHz single element transducer (Olympus) was translated to scan 1D PA images. The RF signal was acquired using an amplifier (AM-1300, MITEQ) and a digital oscilloscope (LeCroy). MRI Samples were scanned with a 3.0T whole-body MRI scanner (Achieva, Philips Healthcare) using a phased array wrist coil. MRIs were obtained using a two-dimensional multislice-multiecho spin echo sequence with various echo times. The imaging parameters were as following: repetition time, 2500 ms; echo times, 10/30/50/70/100 ms; field of view, 10 cm; matrix, 256×256; and thickness, 2 mm. How to cite this article: Jin, Y.D. et al . Multifunctional nanoparticles as coupled contrast agents. Nat. Commun. 1:41 doi: 10.1038/ncomms1042 (2010).